Catalytic N-radical cascade reaction of hydrazones by oxidative deprotonation electron transfer and TEMPO mediation Compared with the popularity of various C-centred radicals, the N-centred radicals remain largely unexplored in catalytic radical cascade reactions because of a lack of convenient methods for their generation. Known methods for their generation typically require the use of N-functionalized precursors or various toxic, potentially explosive or unstable radical initiators. Recently, visible-light photocatalysis has emerged as an attractive tool for the catalytic formation of N-centred radicals, but the pre-incorporation of a photolabile groups at the nitrogen atom largely limited the reaction scope. Here, we present a visible-light photocatalytic oxidative deprotonation electron transfer/2,2,6,6-tetramethylpiperidine-1-oxyl (TEMPO)-mediation strategy for catalytic N-radical cascade reaction of unsaturated hydrazones. This mild protocol provides a broadly applicable synthesis of 1,6-dihydropyradazines with complete regioselectivity and good yields. The 1,6-dihydropyradazines can be easily transformed into diazinium salts that showed promising in vitro antifungal activities against fungal pathogens. DFT calculations are conducted to explain the mechanism. Synthetic chemists continuously strive for fast, selective and high yielding reactions under mild conditions. Radical reactions, especially the radical cascades, provide a potential access to such ideal transformations and have attracted considerable attention of synthetic community because of their typically mild conditions, short reaction times and high efficiency [1] , [2] . Although various carbon radicals have been widely used in catalytic radical-based cascade reactions [3] , [4] , [5] , however, the chemistry of N-centred radicals in this regard remains largely unexplored because of a lack of convenient and general methods for their generation [6] , [7] . Known methods for their generation typically require the use of N-functionalized precursors or various toxic, potentially explosive or unstable radical initiators. Pioneered by Nicolaou’s discovery of the o -iodoxybenzoic acid-mediated conversion of N -aryl amides and carbamates into the corresponding nitrogen radicals [8] , the groups of Chiba [9] and Lei [10] , respectively, developed two efficient methods for the generation of 1,3-diazaallyl and amidyl radicals by Cu- and Ni-catalyzed oxidative cleavage of N–H bonds of amidines and N -alkoxyamides using O 2 and di-tertiary butyl peroxide as terminal oxidants at high temperatures. Recently, Li [11] and Chemler [12] also independently reported the Cu- and Ag-catalyzed oxidative formation of amidyl radicals in the presence of stoichiometric MnO 2 and Selectfluor reagents as oxidants. Despite these impressive advancements, the search for new efficient protocols for direct catalytic conversion of the N–H bonds into the corresponding N-centred radicals under mild conditions has become an increasingly significant, yet challenging priority in the development of new N-radical cascade reactions. In recent years, the visible-light photocatalysis has been established as a powerful technique that facilitates selectively activating organic molecules and chemical bonds to indentify new chemical reactions under mild conditions [13] , [14] , [15] , [16] . As the notable early studies by MacMillan [17] and Sanford [18] on neutral N-centred radical-mediated photocatalytic C–H amination of aldehydes and (hetero)arenes, several promising visible-light photocatalytic protocols have been developed by other groups for generating N-centred radicals and C–N bond formation ( Fig. 1a ) [19] , [20] , [21] , [22] , [23] . Despite their advantages, these methods require the introduction of a photolabile substituent at the nitrogen atom as a handle for photo-activation. The use of the visible-light photocatalysis in initiating strong N–H bond activation and application in neutral N-centred radical-mediated catalytic cascade reactions have been, until recently, very limited. The Knowles’ group recently reported an elegant combination of iridium photocatalyst and phosphate base for a direct homolytic cleavage of strong N–H bonds of N -arylamides to access amidyl radicals by a concerted proton-coupled electron transfer, which allowed an efficient radical cascade reaction towards N-heterocycle synthesis [24] . Exploring new reactivity of N-containing compounds in the field of visible-light photocatalysis is an integral part of our recent ongoing research endeavours [25] , [26] , [27] , [28] . For example, our group has recently developed a direct catalytic conversion of the N–H bonds of β,γ-unsaturated hydrazones into N-centred hydrazonyl radicals by visible-light-induced photoredox catalysis, which enables an efficient and mild approach to intramolecular alkene hydroamination and oxyamination for synthesis of 4,5-dihydropyrazole derivatives [28] . In this reaction, a highly regioselective 5-exo radical cyclization of an N-centred radical was observed. It should be noted that the groups of Han [29] , [30] and Chiba [31] have also independently reported stoichiometric amounts of tetramethylpiperidine-1-oxyl (TEMPO)-mediated intramolecular cyclization of hydrazonyl radicals for pyrazoline synthesis. Inspired by these studies, we considered exploration of the reactivity of hydrazones in catalytic N-radical cascade reactions to assemble biologically and synthetically important dihydropyradazine scaffolds [32] , inaccessible using other thermal methods [29] , [30] , [31] , [33] or our own previous protocols. 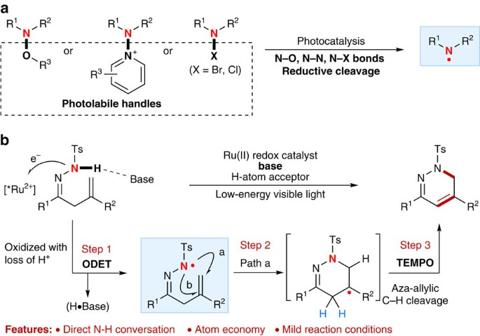Figure 1: Reaction design. (a) Visible-light-induced photocatalytic generation of N-centred radicals from N-functionalized precursors. (b) Our blueprint for catalytic N-radical cascade reaction of hydrazones: merge of oxidative deprotonation electron transfer (ODET) activation of N–H bond with TEMPO mediation. Figure 1: Reaction design. ( a ) Visible-light-induced photocatalytic generation of N-centred radicals from N-functionalized precursors. ( b ) Our blueprint for catalytic N-radical cascade reaction of hydrazones: merge of oxidative deprotonation electron transfer (ODET) activation of N–H bond with TEMPO mediation. Full size image To this end, herein, we report an oxidative deprotonation electron transfer (ODET)/TEMPO-mediation strategy for direct N–H bond activation and catalytic N-radical cascade reactions of unsaturated hydrazones ( Fig. 1b ). This mild protocol represents the first, to our knowledge, broadly applicable synthesis of 1,6-dihydropyradazines with good regioselectivity and yield, achieved by merge of visible-light photocatalysis and TEMPO mediation. Reaction design To realize the target catalytic N-radical cascade reaction of unsaturated hydrazones as shown in Fig. 1b , several major challenges would probably be encountered, such as the controlled formal homolysis of the recalcitrant N–H bond for the formation of the neutral N-centred hydrazonyl radical, regioselectivity of the N-radical cyclization step (for example, 6- endo and 5- exo , path a versus path b) [34] , [35] and selective homolytic activation of aza-allylic C–H bond in C-centred radical intermediate. Notably, it has been recently documented by MacMillan [36] , [37] , Knowles [24] , [38] , [39] and our group [28] , [40] that the addition of a suitable Brønsted acid, Lewis acid or base could facilitate some otherwise inaccessible photocatalytic event by weakening chemical bonds of reactants and co-catalysts or modulating their redox potential. It has also been demonstrated by López and Gómez that complete 6- endo -selectivity over 5- exo ring closure in radical cyclization of C-centred radicals can be controlled by the radical property, substitution pattern at C-5 or ring strain of substrate [34] , [35] . Quite recently, the MacMillan group also first integrated elementary hydrogen atom transfer (HAT) process into H-bond catalysis, and achieved a highly selective photoredox α-alkylation/lactonization cascade of alcohols [41] . Based on these inspiring studies, we hypothesized that the aforementioned regioselective N-radical cascade reaction could possibly be achieved by merging visible-light photoredox with TEMPO-mediated HAT process, wherein the N–H bond might be directly converted into the corresponding N-centred hydrazonyl radical through an ODET and the aza-allylic C–H bond can probably be homolytically cleavaged by a suitable H-atom acceptor such as TEMPO [42] . To test the feasibility of this strategy, we initially conducted density functional theory (DFT) calculations on the cyclization step of N-centred radical intermediates 1a-A , 1b-A and 1c-A with sterically and electronically diverse substituents at the 2-position of the alkene ( Fig. 2a ; see Supplementary Notes 1–3 for details). The energies given in this work are N-12//6-311+G(d, p)//B3 LYP/6-31G(d) calculated Gibbs free energies in chloroform. See the Supplementary Information for more computational details.) [43] . As expected, both 5- exo and 6- endo N-radical-mediated radical cyclizations are possible pathways. For example, the study showed that the 5- exo -trig radical cyclization of 1a-A with an activation free energy of only 8.8 kcal mol −1 via 1a-TS1 is much more favoured than its 6- endo -trig variant (activation free energy of 13.5 kcal mol −1 ; Fig. 1b ). It was also found that 1b-A would undergo 5 -exo cyclization through 1b-TS1 more feasibly than its 6- endo cyclization via 1b-TS2 , as shown by their activation free energy ( Fig. 1c , 7.5 versus 11.2 kcal mol −1 ). Interestingly, the 6- endo cyclization of 1c-A with a phenyl group at the 2-position of the alkene moiety proved to be easier to accomplish through 1c-TS2 , with a relatively low activation free energy of 8.7 kcal mol −1 , to give the C-centred radical intermediate 1c-C ( Fig. 1d ). Encouraged by these computational results, we proceeded to perform experimental studies with these substrates to explore the feasibility of the desired 6- endo radical cyclization. 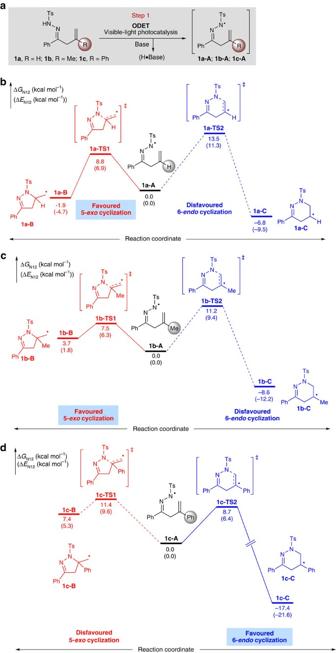Figure 2: Reaction development. (a) Generation of N-radicals by visible-light photocatalysis. (b) Free energy profiles for 5-exoand 6-endoradical cyclizations of1a-A. (c) Free energy profiles for 5-exoand 6-endoradical cyclizations of1b-A. (d) Free energy profiles for 5-exoand 6-endoradical cyclizations of1c-A. Figure 2: Reaction development. ( a ) Generation of N-radicals by visible-light photocatalysis. ( b ) Free energy profiles for 5- exo and 6- endo radical cyclizations of 1a-A . ( c ) Free energy profiles for 5- exo and 6- endo radical cyclizations of 1b-A . ( d ) Free energy profiles for 5- exo and 6- endo radical cyclizations of 1c-A . Full size image Under our previously developed visible-light photocatalytic conditions for hydroamination of β,γ-unsaturated hydrazones [28] , substrates 1a and 1b indeed underwent 5- exo radical cyclization reactions smoothly to give the corresponding products 2a and 2b in 68% and 81% yields, respectively ( Fig. 3a ). These results also provided a solid support for the above computational investigations into these substrates. Interestingly, the reaction of 1c resulted in the formation of a complex mixture with a complete conversion ( Fig. 3b ). Careful analysis of the reaction mixture revealed that an inseparable mixture of products 2c and 3 can be obtained in 21% yield with a ratio of 1:0.9. Meanwhile, product 4 was also isolated in 16% yield, which might be formed through another radical cascade reaction between 1c and the reaction solvent CHCl 3 via radical intermediate 1c-B . The structures of 2a-2c , 3 and 4 were fully characterized by their 1 H and 13 C NMR spectra and mass data, and compound 4 was further characterized by single-crystal X-ray analysis (see Supplementary Fig. 79 for details). Note that the biologically significant 1,6-dihydropyridazines of type 2c cannot be easily prepared using traditional methods [33] . These observations suggested that further optimization of reaction parameters might result in the exclusive formation of the desired 1,6-dihydropyridazines. 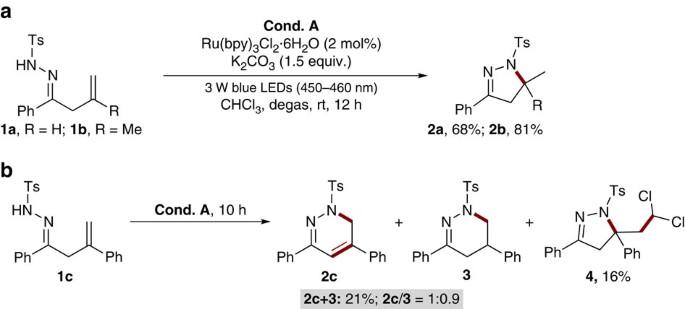Figure 3: Initial results. (a) Reaction of substrate1aand1bunder conditionA. (b) Reaction of substrate1cunder conditionA. Unless otherwise noted, conditionA: reaction were run with1(0.2 mmol), Ru(bpy)3Cl2·6H2O (2mol%), K2CO3(0.3 mmol), 3 W blue light-emitting diodes (450–460 nm) irradiation and CHCl3(4.0 mL) at rt for 10–12 h. Figure 3: Initial results. ( a ) Reaction of substrate 1a and 1b under condition A . ( b ) Reaction of substrate 1c under condition A . Unless otherwise noted, condition A : reaction were run with 1 (0.2 mmol), Ru(bpy) 3 Cl 2 ·6H 2 O (2mol%), K 2 CO 3 (0.3 mmol), 3 W blue light-emitting diodes (450–460 nm) irradiation and CHCl 3 (4.0 mL) at rt for 10–12 h. Full size image Optimization of reaction conditions Encouraged by these initial results, we continued to optimize the reaction conditions with 1c as a model substrate to further improve the selectivity and yield ( Table 1 ). Inspired by the recently demonstrated wide applicability of nitroxides in organic synthesis and their unique properties [44] , [45] , we initially focused on nitroxides as potential additives. Surprisingly, it was found that the addition of TEMPO (1.0 equiv.) did not quench the reaction; instead, it resulted in a clean reaction and gave the desired 1,6-dihydropyridazine 2c in 89% yield (entry 1). Based on our blueprint of the reaction, we postulated that TEMPO might serve as a H-atom acceptor to abstract aza-allylic H-atom by an HAT process [41] . Then, we simply screened inorganic bases such as NaOH, Na 2 CO 3 and Na 2 HPO 4 , and established that the base also played an important role in the reaction, with K 2 CO 3 identified as the best choice (entries 2–4). With K 2 CO 3 as the base, we also briefly examined several other common solvents and CHCl 3 proved to be the best reaction media with tetrahydrofuran, MeOH, dimethylformamide and CH 3 CN giving relatively low yields (entries 5–8). Then, we evaluated the effect of photocatalysts on the reaction under otherwise identical conditions. Interestingly, the use of Ir(ppy) 2 (dtbbpy)PF 6 as a photocatalyst provided comparable results, whereas organic photocatalyst Eosin Y was ineffective for the reaction (entries 9–10). It has been well documented that TEMPO can serve not only as a radical scavenger but also as an oxidant in transition-metal catalysis [44] , [45] . Thus, we continued to test several other oxidants, such as K 2 S 2 O 8 and 2,3-dichloro-5,6-dicyano-1,4-benzoquinone (see Supplementary Table 1 for details). However, all the reactions with these oxidants resulted in a complex mixture without formation of any desired product, suggesting that TEMPO might act as a radical trap to abstract the α-hydrogen atom from intermediate 1c-C to facilitate the target N-radical cascade reaction pathway (entries 11–12). In the control experiments with CHCl 3 or CH 3 CN as the solvent, only very little or no desired products were detected in the absence of photocatalyst, base, TEMPO or light; large amounts of starting materials remained intact, highlighting the critical role of all the parameters in the reaction (entries 13–16; see Supplementary Table 2 for details). Table 1 Optimization of conditions for catalytic N-radical cascade reaction of unsaturated hydrazone 1c . Full size table Substrate scope Under the optimized conditions, we then evaluated the substrate scope of this transformation with a variety of β,γ-unsaturated hydrazones ( Fig. 4 ). First, we examined the effects of arene substitution using a wide range of β,γ-unsaturated hydrazones 1c-1i . It was found that the reaction with various β,γ-unsaturated hydrazones bearing electron-neutral, electron-poor (for example, Cl, Br, CF 3 ) or electron-rich (for example, Me) substituents at the 2-, 3- or 4-position of the aromatic ring proceeded well to deliver the corresponding products 2c - 2i with yields ranging from 61 to 85%. Notably, those aryl bromides are amenable to further synthetic elaborations through transition-metal-catalyzed C–C coupling reactions. Product 2f was also characterized by single-crystal X-ray analysis (see Supplementary Fig. 79 for details). Moreover, 2-naphthyl substituted hydrazone 1j reacted well to afford product 2j in 86% yield. Considering the known medicinal chemistry, it is noteworthy that various heterocycles can be incorporated into the hydrazone substrates with no apparent deleterious effect on the reaction efficiency. For example, 2-thiophenyl and 3-indolyl substituted hydrazones were tolerated well to give the desired products 2k and 2l in 59% and 53% yields, respectively. More importantly, the substrate scope of the current protocol can be successfully extended to aliphatic β,γ-unsaturated hydrazones. Thus, the reaction with a series of linear and branched aliphatic β,γ-unsaturated hydrazones 1m-1r can undergo the radical cascade reaction smoothly under standard conditions, although with prolonged reaction times, to afford the products 2m - 2r in 63–83% yield. The β,γ-unsaturated hydrazone 1s bearing a styryl group also appeared to be viable for the reaction, producing a 70% yield of 2s . Remarkably, cyclic substituents, such as cyclopropyl, cyclopentyl and cyclohexyl groups, could also be easily incorporated into the 1,6-dihydropyridazine scaffold with high yields ( 2t - 2v , 83–96%). 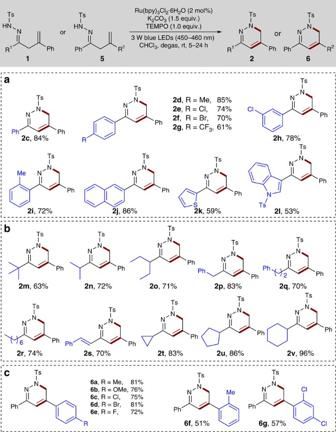Figure 4: Reaction scope of unsaturated hydrazones. (a) Investigation of the effects of arene substitution of hydrazones. (b) Substrate scope of aliphatic unsaturated hydrazones. (c) Substrate scope of alkene moieties. Unless otherwise noted, reactions were run with1or5(0.3mmol), Ru(bpy)3Cl2·6H2O (0.006mmol, 2.0mol%), K2CO3(0.45mmol), TEMPO (0.3mmol) and CHCl3(6.0ml) at rt for 5–24 h under irradiation with 3 W blue light-emitting diodes (450–460 nm). Figure 4: Reaction scope of unsaturated hydrazones. ( a ) Investigation of the effects of arene substitution of hydrazones. ( b ) Substrate scope of aliphatic unsaturated hydrazones. ( c ) Substrate scope of alkene moieties. Unless otherwise noted, reactions were run with 1 or 5 (0.3mmol), Ru(bpy) 3 Cl 2 ·6H 2 O (0.006mmol, 2.0mol%), K 2 CO 3 (0.45mmol), TEMPO (0.3mmol) and CHCl 3 (6.0ml) at rt for 5–24 h under irradiation with 3 W blue light-emitting diodes (450–460 nm). Full size image Encouraged by these results, we proceeded to examine the scope of alkene moieties by incorporation of various substituents into the phenyl ring. As highlighted in Fig. 4c , the substitution patterns and electronic properties of the aromatic ring showed no apparent effect on the reaction efficiency either. For example, all the electron-releasing (for example, 4-Me, 2-Me and 4-MeO) and electron-withdrawing (for example, 4-F, 4-Cl, 4-Br, 2,4-2Cl) groups were well tolerated under the standard conditions, furnishing the expected products 6a-6g in 51–81% yield. Interestingly, during our subsequent biological studies with 1,6-dihydropyridazines 2- and 6 -derived diazinium salts, it was found that such aromatic substituents at the 2-position of the alkene are critical to their antifungal in vitro activities. It should be noted that we did not detect any 5- exo cyclization products in all cases [29] , [30] . Mechanistic investigations To gain additional insights into the reaction mechanism, several control experiments were conducted with model substrate 1c ( Fig. 5 ; see Supplementary Discussion for details). To further confirm the formation of C-centred intermediate of type 1c - C during the reaction, common radical trapping agents (PhSeSePh or 2,6-di-tert-butyl-4-methylphenol, BHT) were added to the reaction system to capture the radical intermediate ( Fig. 5a ). However, no trapping products were observed; instead, only the 1,6-dihydropyridazine 2c was produced and isolated in 85% and 83% yields, respectively. In contrast, without addition of TEMPO, the reaction with PhSeSePh as a radical trapping agent furnished a mixture of desired 2c and selenide-adduct 7 (61% yield, 1:4 ratio; see Supplementary Fig. 78 for details), and compound 7 should be formed from radical intermediate 1c - C and PhSeSePh ( Fig. 5b ). Then, we obtained the pure selenide-adduct 7 by semi-preparative high-performance liquid chromatography purification and re-subjected it to the standard reaction conditions without TEMPO ( Fig. 5c ). However, we did not detect any desired product 2c even after 24 h and compound 7 remained intact, suggesting that selenide-adduct 7 should not be the possible intermediate for the formation of 1,6-dihydropyridazine 2c . 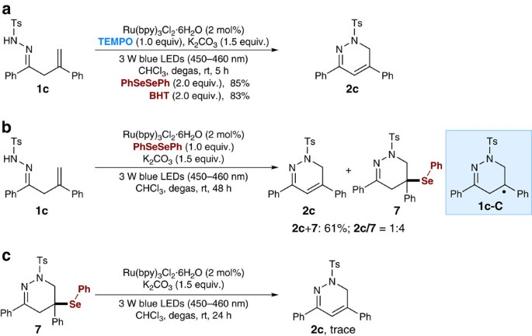Figure 5: Mechanistic investigations. (a) Trapping the C-centred intermediate by addition of PhSeSePh or BHT under the standard conditions. (b) Trapping the C-centred intermediate by addition of PhSeSePh under the standard conditions in the absence of TEMPO. (c) Control experiment with selenide-adduct7under the standard conditions. Figure 5: Mechanistic investigations. ( a ) Trapping the C-centred intermediate by addition of PhSeSePh or BHT under the standard conditions. ( b ) Trapping the C-centred intermediate by addition of PhSeSePh under the standard conditions in the absence of TEMPO. ( c ) Control experiment with selenide-adduct 7 under the standard conditions. Full size image To further determine the role of TEMPO, we also calculated the free energy of the subsequent transformation of C-centred radical intermediate 1c - C into the final product 2c via the minimum energy crossing point (MECP; Fig. 6 ) [43] . As shown in Fig. 6a , the computational results showed that the TEMPO might facilitate the conversion of the intermediate 1c - C into the final product 2c through a TEMPO-mediated HAT process, because the calculated energy barrier (Δ E ) for the aza-allylic hydrogen atom abstraction via MECP-I is only 18.8 kcal mol −1 . Moreover, the generation of product 2c is exergonic by 20.0 kcal mol −1 compared with the intermediate 1c - C . Recently, a similar trapping of carbon radical and elimination of TEMPO-H process in the presence of base has been identified by Chiba’s group as the possible pathway in TEMPO-mediated C–H bond oxygenation of oximes and hydrazones [46] . Inspired by this work, another possible pathway involving carbon radical trapping/elimination sequence of 1c - C in the presence of base was also considered in calculation. As shown in Fig. 6b , the combination of radical 1c - C with TEMPO occurs through MECP-II , and the energy barrier (Δ E ) of which is 18.4 kcal mol −1 . Although this energy barrier is close to that of MECP-I formation ( Fig. 6a ), the formation of TEMPO-adduct 8 is endergonic by 19.3 kcal mol −1 compared with 1c - C . Moreover, the activation free energy of subsequent deprotonation, which occurs via transition state 9-TS , reaches as high as 43.3 kcal mol −1 . According to these results, the sequential combination of carbon radical 1c - C with TEMPO and elimination process appears to be thermodynamically unfavourable. Moreover, we also intended to isolate the possible intermediate 8 upon ∼ 50% conversion of model substrate 1c . Unfortunately, all the attempts met failure, although a trace amount of intermediate 8 was detected by the high-resolution mass spectrometry analysis of the the reaction mixture (see Supplementary Information). Another possible pathway for base-free elimination of TEMPO-H from 8 by direct radical elimination with C–O bond homolysis is not considered as the stoichiometric base is necessary in our reaction system [47] , [48] , [49] . Taken together, although the calculation studies support the TEMPO-mediated HAT process as the likely mechanism for the transformation of C-centred radical intermediate 1c - C into the final product 2c , at present we cannot rule out the carbon radical recombination/elimination pathway (see Supplementary Figs 80 and 81 and Supplementary Notes 1-3 for details). More detailed mechanistic studies are curently underway in our laboratory. 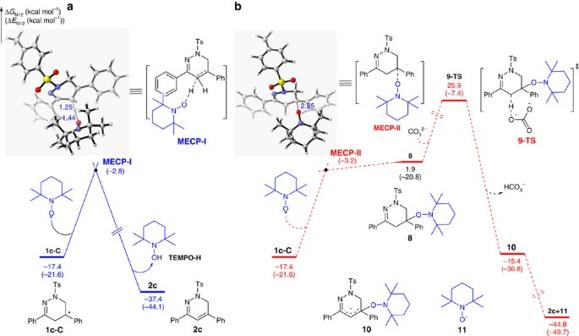Figure 6: Calculation studies. (a) Free energy profile for the transformation of C-centred radical1c-Cinto product2cthrough a TEMPO-mediated HAT process. (b) Free energy profile for the transformation of C-centred radical1c-Cinto product2cthrough carbon radical trapping/elimination process. Figure 6: Calculation studies. ( a ) Free energy profile for the transformation of C-centred radical 1c-C into product 2c through a TEMPO-mediated HAT process. ( b ) Free energy profile for the transformation of C-centred radical 1c-C into product 2c through carbon radical trapping/elimination process. Full size image According to our blueprint for ODET activation of N–H bond, the addition of K 2 CO 3 proved be critical for the reaction as a base and this phenomenon was indeed observed during the optimization study ( Table 1 , entry 14). To further evaluate the role of base in these reactions, we continue to study the mechanism of N-centred hydrazonyl radical formation by luminescence quenching experiments, NMR and electrochemical analysis with 1c as a model substrate (see Supplementary Figs 82–86 for details). Stern–Volmer analysis demonstrated that hydrazone 1c alone is unable to quench the excited state of *[Ru(bpy) 3 ] 2+ in dimethylformamide at 25 °C, implying that the excited state ruthenium complex does not oxidize the hydrazone 1c directly. However, upon addition of K 2 CO 3 as a base, a significant decrease of luminescence emission intensity was observed. In addition, the 1 H NMR analysis of a solution containing both 1c and K 2 CO 3 exhibited that the addition of K 2 CO 3 resulted in complete disappearance of the signal of N–H, suggesting that K 2 CO 3 serve to abstract the proton of N–H bond to generate nitrogen anion intermediate 1c’ ( Fig. 7 and Supplementary Information). Moreover, cyclic voltammetry data confirmed that the excited photocatalyst *Ru(bpy) 3 2+ ( E 1/2 *II/I =+0.77 V versus SCE in CH 3 CN) is likely to be sufficiently oxidizing to oxidize the nitrogen anion 1c’ ( E p red =0.56 V versus SCE) to generate the corresponding N-centred radical intermediate 1c-A ( Fig. 7 ). Taken together, although we could not completely exclude the concerted proton-coupled electron transfer mechanism at the current stage [24] , [38] , [39] , the above results are more consisted with an ODET activation mechanism involving sequential deprotonation of hydrazone substrates by the K 2 CO 3 and visible-light photocatalytic single-electron transfer (SET) oxidation. 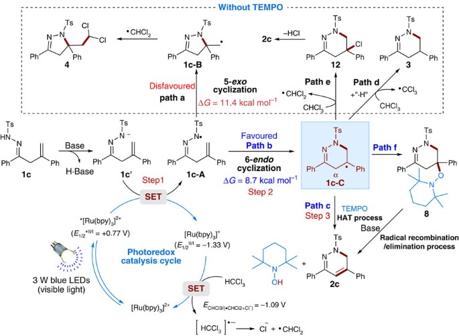Figure 7: Proposed catalytic cycle. The plausible mechanism involves oxidative deprotonation electron transfer (ODET) activation of N–H bond into N-centred radical by visible light photoredox catalysis and TEMPO-mediated N-radical cyclization. Figure 7: Proposed catalytic cycle. The plausible mechanism involves oxidative deprotonation electron transfer (ODET) activation of N–H bond into N-centred radical by visible light photoredox catalysis and TEMPO-mediated N-radical cyclization. Full size image Ultimately, a plausible mechanism is outlined in Fig. 7 using 1c as an example. Initially, the β,γ-unsaturated hydrazone 1c is transformed into anionic intermediate 1c’ upon deprotonation, which is then oxidized to the N-centred radical 1c - A by the excited photocatalyst *[Ru(bpy) 3 ] 2+ through a SET process. Then, the key intermediate 1c - A undergoes a 6- endo radical cyclization to afford the C-centred benzylic radical intermediate 1c - C , which can be conveniently transformed into the final product 2c by an HAT process in the presence of TEMPO (path c). However, as for the transformation of C-centred radical intermediate 1c-C into the final product 2c , at the current stage, we cannot rule out the carbon radical recombination/elimination pathway that involves TEMPO-adduct 8 as the key intermediate (path f, see Supplementary Information). In the absence of TEMPO, the intermediate 1c - C can abstract a hydrogen atom directly from CHCl 3 to give 1,4,5,6-tetrahydropyridazine 3 (path d). Meanwhile, the intermediate 1c - C can also abstract a chlorine radical from chloroform to give rise to dichloromethyl radical and labile tertiary chloride adduct 12 intermediate [50] , which can undergo facile elimination to give the product 2c . Moreover, without addition of TEMPO, the intermediate N-centred radical 1c - A could also undergo a 5- exo radical cyclization (path a) to furnish 1c - B , partly because of the relatively small activation free energy difference between 1c - B and 1c - C ( Fig. 2d ). In the photocatalytic cycle, chloroform can regenerate the photocatalyst [Ru(bpy) 3 ] 2+ by an SET oxidation process with the concomitant release of the chloroform radical anion, which rapidly dechlorinated to give chloride ion and the dichloromethyl radical [51] , [52] , [53] , [54] . The formation of a dichloromethyl radical in the reaction was also confirmed by the isolation of side product 4 , resulting from the radical cross coupling between the dichloromethyl radical and 1c - B intermediate. Synthetic application To further demonstrate the synthetic potential of this method, a gram-scale reaction of β,γ-unsaturated hydrazone 1c was conducted in the presence of 1 mol% of photocatalyst under standard reaction conditions, and the desired product 2c was still successfully obtained in 74% yield after 48 h ( Fig. 8a ). A key benefit of this photocatalytic radical cyclization strategy is that the β,γ-unsaturated hydrazone starting materials are easily accessed from the corresponding β,γ-unsaturated ketones and tosyl hydrazine. Thus, we examined the photocatalytic radical cyclization with β,γ-unsaturated ketone 13 and tosyl hydrazine in a two-step one-pot process ( Fig. 8b ). Pleasingly, the desired 1,6-dihydropyridazine 2d was obtained in 67% overall yield. Recently, heteroaromatic N -oxides have been widely employed in transition-metal-catalyzed aromatic C–H activation/functionalization reactions to access various valuable heterocyclic molecules [55] . We found that the present method could provide a new approach to the synthesis of pyridazine N -oxides. For example, treatment of 2c with m -CPBA as the oxidant resulted in the facile formation of pyridazine N -oxide 14 in a 70% yield that was also clearly determined by X-ray analysis ( Fig. 8c ; see Supplementary Fig. 79 for details). 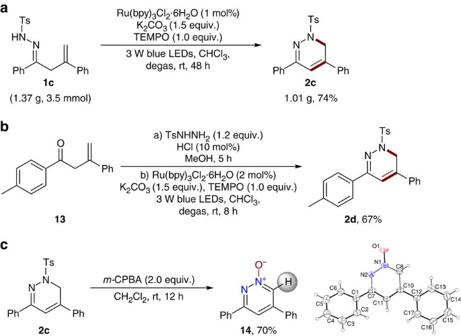Figure 8: Synthetic application. (a) Gram-scale reaction. (b) One-pot process for synthesis of 1,6-dihydropyridazine2d. (c) Synthesis of pyridazineN-oxide14. Figure 8: Synthetic application. ( a ) Gram-scale reaction. ( b ) One-pot process for synthesis of 1,6-dihydropyridazine 2d . ( c ) Synthesis of pyridazine N -oxide 14 . Full size image Moreover, it was then established that the 1,6-dihydropyridazine products can also be easily transformed into the corresponding biologically important pyridazines under mild conditions (2.0 equiv. NaOH in CH 3 CN at 80 °C). As highlighted in Fig. 9a , the electronic and steric properties of the substituents on both of the aromatic rings showed no significant effect on the reaction efficiency. A series of substrates with electron-rich or electron-poor substituents worked well to give the desired products in good yields ( 15a - 15d , 86–90% yield; 15i – 15l , 81–89% yield). In addition, 2-thiophenyl and 2-naphthyl-substituted 1,6-dihydropyridazines reacted well to give the corresponding pyridazine products 15d and 15e in 90% and 94% yield, respectively. Remarkably, the 1,6-dihydropyridazines bearing alkyl groups such as isopropyl, tert -butyl and cyclohexyl substituents, were well tolerated to deliver the desired products 15f-15h in high yields (76–87%). 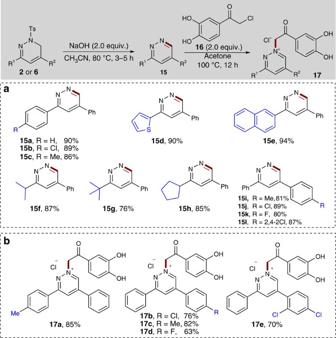Figure 9: Application to the synthesis of pyridazines and diazinium salts. (a) Reactions were run with2or6(0.2 mmol), NaOH (0.6 mmol) and CH3CN (4.0 ml) at 80 °C for 3–5 h. (b) Reactions were run with15(0.3 mmol),16(0.6 mmol) and acetone (3.0 ml) at 100 °C for 12 h. Figure 9: Application to the synthesis of pyridazines and diazinium salts. ( a ) Reactions were run with 2 or 6 (0.2 mmol), NaOH (0.6 mmol) and CH 3 CN (4.0 ml) at 80 °C for 3–5 h. ( b ) Reactions were run with 15 (0.3 mmol), 16 (0.6 mmol) and acetone (3.0 ml) at 100 °C for 12 h. Full size image It has recently been documented that the pyridazine derivatives, such as diazinium salts bearing a dihydroxyacetophenone core, showed promising biological activities against a variety of microorganisms (germs and fungi) [56] . Thus, we further attempted to transform a range of representative pyridazines 15 into the corresponding diazinium salts 17 and preliminarily explored their potential structure–activity relationships ( Fig. 9b ). By refluxing a mixture of pyridazines 15 and 2-chloro-3′,4′-dihydroxyacetophenone 16 in acetone for 12 h, a series of diazinium salts 17a - 17e were easily obtained in 63–85% yield after a simple filtration. Over the past decades, the incidence of invasive fungal infections and the associated morbidity and mortality rates have risen remarkably due to the over-use of broad-spectrum antibiotics, serious medical interventions and immune deficiency disorders, such as AIDS [57] , [58] . Despite recent additions to the antifungal drug family, the limitations of the current antifungal drugs involve narrow activity spectra, detrimental drug–drug interactions and antifungal resistance, necessitating the development of new antifungal agents or leads. With diazinium salts 17a - 17e in hand, we evaluated the in vitro antifungal activities of these compounds against eight human pathogenic fungi, compared with commercially available fluconazole. In contrast to the antibacterial activities reported for related diazinium salts [56] , our results demonstrated that some of these compounds showed promising activities against four common clinical pathogenic fungi ( Candida albicans , C. parapsilosis , C. neoformans and C. glabrata ; see Supplementary Tables 3 and 4 for details). These results also confirmed that the substitution patterns and electronic properties of the substituents at both of the phenyl rings are critical to their in vitro antifungal activities. Gratifyingly, the MIC 80 values of most of the compounds ( 17b - 17e ) against C. parapsilosis , C. neoformans and C. glabrata (0.5–4 μg ml −1 ) were comparable to those of fluconazole, which should be valuable for our future biological studies. We have developed a novel ODET/HAT strategy, which we used to directly convert the N–H bond of β,γ-unsaturated hydrazones to the N-centred radical, and developed an efficient catalytic N-radical cascade reaction. This mild protocol represents the first, to our knowledge, broadly applicable synthesis of 1,6-dihydropyradazines with good regioselectivity and yield, achieved by the merge of visible-light photocatalysis and TEMPO mediation. The 1,6-dihydropyridazines could also be conveniently transformed into biologically important diazinium salts bearing dihydroxyacetophenone core, which showed promising antifungal in vitro activities against various fungal pathogens. Control experiments and DFT calculations have been performed to help explain the mechanism. Owing to the wide occurrence of various N–H bonds, we believe that this strategy may find wide use for generation of other various N -centred radicals and new reaction developments with these reactive species [59] . Materials Unless otherwise noted, materials were purchased from commercial suppliers and used without further purification. All the solvents were treated according to general methods. Flash column chromatography was performed using 200–300 mesh silica gel. The manipulations for photocatalytic N-radical cascade reactions were carried out with standard Schlenk techniques under Ar by visible-light irradiation. See Supplementary Methods for experimental details. General methods 1 H NMR spectra were recorded on 400 or 600 MHz spectrophotometers. Chemical shifts are reported in delta ( δ ) units in parts per million (p.p.m.) relative to the singlet (0 p.p.m.) for tetramethylsilane. Data are reported as follows: chemical shift, multiplicity (s=singlet, d=doublet, t=triplet, dd=doublet of doublets, m=multiplet), coupling constants (Hz) and integration. 13 C NMR spectra were recorded on 100 or 150 MHz with complete proton-decoupling spectrophotometers (CDCl 3 : 77.0 p.p.m. or DMSO-d 6 : 39.5 p.p.m.). 19 F NMR spectra were recorded on 376 MHz with complete proton-decoupling spectrophotometers. Mass spectra were measured on MS spectrometer (EI) or liquid chromatography-mass spectrometry (LC/MS), or electrospray ionization mass spectrometry (ESI-MS). High-resolution mass spectrometry was recorded on Bruker ultrafleXtreme matrix-assisted laser desorption/ionization–time-of-flight (TOF)/TOF mass spectrometer. 1 H NMR, 13 C NMR and 19 F NMR spectra are supplied for all compounds: see Supplementary Figs 1–77 . General procedure for catalytic nitrogen radical cascade reaction of hydrazones In a flame-dried Schlenk tube under Ar, 1c (117.0 mg, 0.3 mmol), Ru(bpy) 3 Cl 2 .6H 2 O (0.006 mmol), TEMPO (46.9 mg, 0.3 mmol) and K 2 CO 3 (61.2 mg, 0.45 mmol) were dissolved in CHCl 3 (6.0 ml). Then, the resulting mixture was degassed via ‘freeze-pump-thaw’ procedure (three times). After that, the solution was stirred at a distance of ∼ 5 cm from a 3-W blue light-emitting diodes (450–460 nm) at room temperature ∼ 5 h until the reaction was completed as monitored by thin-layer chromatography analysis. The crude product was purified by flash chromatography on silica gel (petroleum ether/ethyl acetate 20:1 ∼ 10:1) directly to give the desired product 2c in 84% yield as a white solid. Full experimental details and characterization of new compounds can be found in the Supplementary Methods . Accession codes: The X-ray crystallographic coordinates for structures reported in this Article have been deposited at the Cambridge Crystallographic Data Centre (CCDC), under deposition numbers CCDC 1407651 (2 f), 1407652 (4), 1407653 (14). These data can be obtained free of charge from the Cambridge Crystallographic Data Centre via http://www.ccdc.cam.ac.uk/data_request/cif . How to cite this article: Hu, X.-Q. et al . Catalytic N-radical cascade reaction of hydrazones by oxidative deprotonation electron transfer and TEMPO mediation. Nat. Commun. 7:11188 doi: 10.1038/ncomms11188 (2016).